Nanoparticle-formulated siRNA targeting integrins inhibits hepatocellular carcinoma progression in mice Integrins play an important role during development, regulating cell differentiation, proliferation and survival. Here we show that knockdown of integrin subunits slows down the progression of hepatocellular carcinoma (HCC). Using nanoparticulate delivery of short interfering RNAs targeting β1 and αv integrin subunits, we downregulate all integrin receptors in hepatocytes. Short-term integrin knockdown (2 weeks) does not cause apparent structural or functional perturbations of normal liver tissue. Alterations in liver morphology accumulate on sustained integrin downregulation (7 weeks). The integrin knockdown leads to significant retardation of HCC progression, reducing proliferation and increasing tumour cell death. This tumour retardation is accompanied by reduced activation of the MET oncogene as well as expression of its mature form on the cell surface. Our data suggest that transformed proliferating cells from HCC are more sensitive to knockdown of integrins than normal quiescent hepatocytes, highlighting the potential of small interfering RNA-mediated inhibition of integrins as an anti-cancer therapeutic approach. Integrins are extracellular matrix (ECM) receptors that play important and diverse roles in metazoans, including regulation of cell motility, differentiation, survival and proliferation [1] . Two ubiquitously expressed families of integrins are formed by dimerization of either the β1 integrin subunit (Itgb1) with one of 12 alpha subunits or the αv integrin subunit with one of β1, β3, β5, β6 or β8 subunits [1] , [2] . The cytoplasmic domain of Itgb1 interacts with multiple proteins and transmits outside signals to cytoskeleton proteins and various membrane receptors. In vivo studies have demonstrated the importance of Itgb1 for early stages of embryonic development. Tissue-specific depletion of Itgb1 in cartilage as well as different epithelial tissues, such as mammary gland and skin, negatively affected cell survival and proliferation in these tissues [3] , [4] , [5] , [6] , [7] , [8] , [9] . A critical role of Itgb1 for liver (and endoderm-derived tissues) formation has been shown in experiments with chimeric mice, where Itgb1-null cells did not participate in liver formation [3] . Whereas the role of integrins in proliferating cells and developing tissues is well established, their role in mature, adult tissues with low proliferation rates (such as brain, kidney, heart and liver) has been less studied. It is assumed that outside-in signalling from the ECM is also required for cell survival in these tissues. This assumption is also based on a number of studies demonstrating a key role of integrins in cell survival and proliferation in vitro [10] , [11] . However, the requirement of Itgb1 in cell and tissue homeostasis is not well understood. Hepatocellular carcinoma (HCC) is the third leading cause of cancer-related deaths worldwide with >600,000 new incidents per year [12] . At diagnosis, most of the patients present with advanced HCC, multiple tumour nodules and have a poor prognosis. To date, sorafenib is the only approved first-line therapeutics for the advanced disease, which only modestly extends overall survival time [13] . However, no curative second-line treatment of HCC has been found. A role of the MET proto-oncogene has been well established in tumour development and metastatic progression. The efficacy of MET inhibitors has been confirmed in preclinical and phase II clinical studies [14] . The cell-matrix adhesion has been shown to be important for MET activity in hepatoma cells isolated from MET-induced liver cancer [15] . Given that most HCC patients present with cirrhosis and thus significant ECM remodelling, targeting cell adhesion receptors can be a promising option in management of liver cancer. The role of interactions of tumour cells with the ECM in the initiation and progression of cancer is contradictory. On one hand, most tumour-derived epithelial cells survive in the absence of adhesion (anchorage-independent proliferation), on the other hand, integrins, including Itgb1 and Itgav, are known to be crucial for proliferation of tumour cells [2] , [16] , [17] , [18] . Upregulation of Itgb1 expression enhances cancer cell viability by promoting survival and conferring resistance to chemotherapy [19] , [20] . An activating mutation of Itgb1 increases conversion of benign tumours to malignant ones in skin [21] . Studies with blocking antibodies against Itgb1 also support its important role in tumourigenesis in breast cancer models [22] . Here we investigate the role of integrins in normal hepatocytes in adult mice by using an in vivo RNA interference (RNAi) approach to specifically reduce integrin expression in liver; this method allows direct comparison of the requirement of integrins for normal and transformed hepatocytes in the same tissue-specific context [23] . We have found that deep knockdown of integrins (particularly, >90% downregulation of integrin receptors comprised of the β1 subunit) in liver parenchymal cells leads to barely detectable alterations during the first 2–4 weeks of knockdown; changes in hepatocyte morphology become apparent by 7 weeks of treatment with Itgb1-specific small interfering RNA (siRNA), while no apparent signs of cell death and/or tissue failure are detected. The development of spontaneous MET/β-catenin-driven HCC is critically dependent on normal levels of integrins in tumour cells. 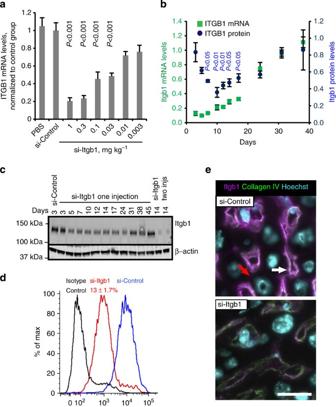Figure 1: RNAi-mediated hepatic silencing of Itgb1. (a) Dose-dependent Itgb1 mRNA knockdown 3 days after siRNA injection(n=4–5, mean±s.e.m.,P-levels—comparison to the si-Control-treated group by the Turkeypost hoctest, (b) time-course of Itgb1 knockdown on the mRNA and protein level after a single dose of siRNA (0.5 mg kg−1,n=3).P<0.001 for mRNA levels in si-Itgb1-treated animals (time points, 3–24 days compared with si-control-treated animals by the Turkeypost hoctest.P-levels on the graph for comparison of Itgb1 protein level with si-control-treated animals by the Turkeypost hoctest. (c) Representative western blot of the time-course. (d) Analysis by flow cytometry of the Itgb1 expression on hepatocytes isolated from animals treated twice with Itgb1 siRNA. (±1° Ab—isotype control/primary antibodies added). Number indicates geometry mean of fluorescent intensity of si-Itgb1-treated cells normalized to one of the control group and represented as mean±s.e.m. For extensive analysis of expression of other integrin subunits, their quantificationSupplementary Fig. 2and for mRNA knockdown quantification seeSupplementary Fig. 2d. (e) Analysis of Itgb1 expression by immunofluorescent staining, expression on hepatocytes (red arrows, lateral surface and white arrow, basal surface). Scale bar, 20 μm. Hepatocyte-specific Itgb1 knockdown in mouse liver Messenger RNA (mRNA) of two β-subunits of integrin, namely β1 and β5, and four α-subunits: Itga1, Itga5, Itga9 and Itgav, were detected in freshly isolated mouse hepatocytes by quantitative PCR (qPCR) ( Supplementary Table 1 ). Itgb1, Itga5 and Itgav were also detected in a HCC cell line grown on collagen at similar levels. To investigate the role of integrin subunits in hepatocytes in liver, we used chemically modified siRNA formulated into lipidoid-based nanoparticles (LNP), which primarily target hepatocytes [24] . Specific siRNAs against mRNAs of interest were selected ( Supplementary Fig. 1a–g ) as previously described [24] , [25] , [26] . Maximal knockdown of Itgb1 mRNA level (80–85%) in vivo , tested at 72 h post injection, was observed at doses ⩾ 0.3 mg kg −1 ( Fig. 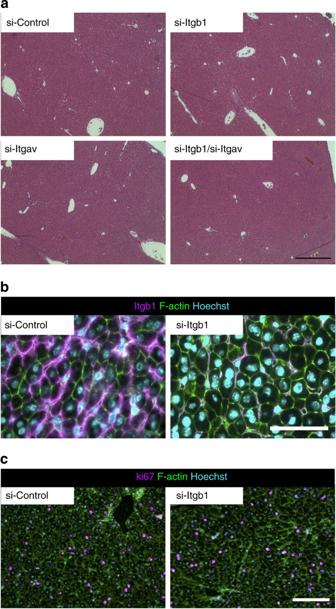Figure 2: Histological analysis of livers after knockdown of integrins in adult and growing mice. (a) Eight–week-old animals received two injections (once per week) of 0.5 mg kg−1of each specific siRNA. Control animals received 1.0 mg kg−1of control siRNA, doses in the groups si-Itgb1 and si-Itgav were adjusted with 0.5 mg kg−1of control siRNA. Animals were euthanized 7 days after the last injection. Haematoxylin eosin staining of the liver sections. Scale bar, 400 μm (b,c). Immature mice received six intraperitoneal injections of si-Itgb1 starting 7 days after birth, twice per week. (b) Immunofluorescent analysis of Itgb1 knockdown. Scale bar, 50 μm. (c) Immunofluorescent analysis of hepatocyte proliferation, staining for Ki67. Scale bar, 100 μm. 1a , detailed description of experiments is presented in Supplementary Table 2 ). The knockdown of Itgb1 was liver specific ( Supplementary Fig. 1h , see also accompanying manuscript of Speicher et al. [27] for other tissues). Maximal mRNA silencing was achieved after 1 day and lasted at least 10 days, followed by a slow recovery. Sixty per cent of Itgb1 protein reduction was observed 10 days after a single injection of siRNA ( Fig. 1b,c ). To achieve 80% knockdown of Itgb1 protein, we performed two weekly injections of siRNA (14 days), Fig. 1c , right). Moreover, we found 90% reduction in protein and mRNA in hepatocytes isolated from liver after treatment with Itbg1-specific siRNA ( Fig. 1d ; Supplementary Fig. 2 ). Slower knockdown of Itgb1 protein in vivo vs in vitro can likely be explained by prevalence of the maturely glycosylated stable form of Itgb1 in hepatocytes [28] . Residual levels of Itgb1 can be at least partially explained by its expression in non-parenchymal cells. Immunofluorescent analysis of liver sections confirmed significant reduction in the Itgb1 expression on hepatocytes ( Fig. 1e ). We validated the RNAi mechanism of Itgb1 mRNA downregulation using 5′-RACE. A predicted cleavage site was identified exclusively in Itgb1-specific siRNA-treated liver samples ( Supplementary Fig. 3a,b ). Figure 1: RNAi-mediated hepatic silencing of Itgb1. ( a ) Dose-dependent Itgb1 mRNA knockdown 3 days after siRNA injection( n =4–5, mean±s.e.m., P -levels—comparison to the si-Control-treated group by the Turkey post hoc test, ( b ) time-course of Itgb1 knockdown on the mRNA and protein level after a single dose of siRNA (0.5 mg kg −1 , n =3). P <0.001 for mRNA levels in si-Itgb1-treated animals (time points, 3–24 days compared with si-control-treated animals by the Turkey post hoc test. P -levels on the graph for comparison of Itgb1 protein level with si-control-treated animals by the Turkey post hoc test. ( c ) Representative western blot of the time-course. ( d ) Analysis by flow cytometry of the Itgb1 expression on hepatocytes isolated from animals treated twice with Itgb1 siRNA. (±1° Ab—isotype control/primary antibodies added). Number indicates geometry mean of fluorescent intensity of si-Itgb1-treated cells normalized to one of the control group and represented as mean±s.e.m. For extensive analysis of expression of other integrin subunits, their quantification Supplementary Fig. 2 and for mRNA knockdown quantification see Supplementary Fig. 2d . ( e ) Analysis of Itgb1 expression by immunofluorescent staining, expression on hepatocytes (red arrows, lateral surface and white arrow, basal surface). Scale bar, 20 μm. Full size image We have validated using qPCR analysis that none of the mRNA of integrin subunits was significantly overexpressed in the hepatocytes isolated from livers treated with siRNA against Itgb1. Using flow cytometry, we confirmed that α1 and α5 integrin subunit levels were lowered on the surface of hepatocytes isolated from animals treated with si-Itgb1, similar observation was done using HCC cells treated with si-Itgb1 in vitro . In contrast, integrin αv subunit was upregulated in both cases ( Supplementary Fig. 2 ). Itgb1 expression may regulate subcellular localization and stability of alpha v integrins, e.g., loss of Itgb1 expression in embryonic stem cells leads to αv integrin re-localization at cell surface and in focal contacts [29] , [30] . The effect of integrin knockdown in liver Treatment with Itgb1 siRNA for 2 weeks did not induce significant morphological changes in livers ( Fig. 2a ). We also did not find changes in serum chemistry, including levels of transaminases, albumin and lipid profile ( Table 1 ). Moreover, continuous inhibition of Itgb1 expression starting from the second week after mouse birth did not inhibit liver growth (liver/body mass ratio of treated animals was not different from controls, and numbers of Ki67-positive cells were not reduced) ( Fig. 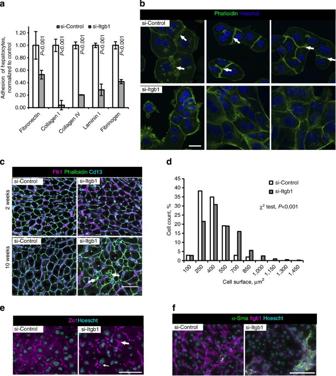Figure 3: Itgb1 knockdown regulates hepatocytes adhesion and morphologyin vivoandex vivo. (a) Downregulation of Itgb1 decreases adhesion of isolated hepatocytes to extracellular matrix proteinsex vivo(n=3). (b) Downregulation of Itgb1 in hepatocytes affects ability of hepatocytes to restore their polarityex vivo. Arrows indicate intercellular space (apical domains) reformed in hepatocytes when cultured in a collagen sandwich. Three independent fields are presented for each treatment. Scale bar, 20 μm. (a,b) Hepatocytes were isolated from mice treated with si-Itgb1 for 10 days (two injections). (c) Long-term silencing of Itgb1 leads to distortion of hepatocyte apical domains (bile canaliculi)in vivo, visualized by Cd13 localization (arrowheads). Subpopulation of enlarged hepatocytes (asterisks) is significantly expanded. Scale bar, 50 μm. (d) Distribution of hepatocyte cell surface in animals treated with si-Itgb1 for 10 weeks. Cell surface was assessed on phalloidin-stained liver sections (~100 cells per animal) using ImageJ software (n=4 per group). (e) Effect of long-term (10 weeks) knockdown of Itgb1 on hepatocyte apical domains (canaliculi) in adult mice treated with si-Itgb1 for 10 weeks. Arrows indicate distorted canaliculi. Scale bar, 50 μm. (f) Increased abundance of activated stellate cells evidenced by immunofluorescent staining for α-smooth muscle actin (α-Sma). Scale bar, 100 μm. 2b,c ) and did not induce significant hepatic toxicity as evidenced by levels of transaminases in serum ( Supplementary Table 3 ). To test the effect of knockdown of all integrin subunits on liver tissue integrity, we developed siRNA against Itgav comprising the second group of hepatic integrin receptors ( Supplementary Figs 1g and 2 ). We did not observe any changes in tissue morphology or serum chemistry in animals treated for 2 weeks with either the combination of siRNA against Itgb1 and Itgav or in the animals treated with individual siRNAs ( Table 1 ; Fig. 2a ). Figure 2: Histological analysis of livers after knockdown of integrins in adult and growing mice. ( a ) Eight–week-old animals received two injections (once per week) of 0.5 mg kg −1 of each specific siRNA. Control animals received 1.0 mg kg −1 of control siRNA, doses in the groups si-Itgb1 and si-Itgav were adjusted with 0.5 mg kg −1 of control siRNA. Animals were euthanized 7 days after the last injection. Haematoxylin eosin staining of the liver sections. Scale bar, 400 μm ( b , c ). Immature mice received six intraperitoneal injections of si-Itgb1 starting 7 days after birth, twice per week. ( b ) Immunofluorescent analysis of Itgb1 knockdown. Scale bar, 50 μm. ( c ) Immunofluorescent analysis of hepatocyte proliferation, staining for Ki67. Scale bar, 100 μm. Full size image Table 1 Effect of short-term knockdown of integrins in mouse liver on parameters of serum chemistry. Full size table One possible interpretation of these results is that the partial, although deep (~90%), knockdown of integrins may not be sufficient to alter the function of hepatocytes within the tissue or may be compensated by other ECM receptors. Therefore, we isolated primary hepatocytes from normal and knockdown liver and tested their adhesion properties in vitro . The reduction of the β1 subunit strongly inhibited the adhesion of hepatocytes isolated from mouse to selected matrices, especially to collagens I and IV ( Fig. 3a ). We also tested whether Itgb1 reduction had an effect on hepatocyte polarity like in other epithelial cells [31] . Primary hepatocytes can re-establish cell polarity and cell–cell contacts when cultured in a double layer of collagen [24] , [32] . Control hepatocytes were able to polarize, forming apical domains and structures resembling bile canaliculi. In contrast, cells with reduced levels of Itgb1 did not form such structures, as visualized by disposition of F-actin filaments ( Fig. 3b ). These results suggest that the function of integrins is necessary under conditions where hepatocytes are outside of the tissue context and forced to re-establish cell–ECM interactions and polarity in vitro . Figure 3: Itgb1 knockdown regulates hepatocytes adhesion and morphology in vivo and ex vivo. ( a ) Downregulation of Itgb1 decreases adhesion of isolated hepatocytes to extracellular matrix proteins ex vivo ( n =3). ( b ) Downregulation of Itgb1 in hepatocytes affects ability of hepatocytes to restore their polarity ex vivo . Arrows indicate intercellular space (apical domains) reformed in hepatocytes when cultured in a collagen sandwich. Three independent fields are presented for each treatment. Scale bar, 20 μm. ( a , b ) Hepatocytes were isolated from mice treated with si-Itgb1 for 10 days (two injections). ( c ) Long-term silencing of Itgb1 leads to distortion of hepatocyte apical domains (bile canaliculi) in vivo , visualized by Cd13 localization (arrowheads). Subpopulation of enlarged hepatocytes (asterisks) is significantly expanded. Scale bar, 50 μm. ( d ) Distribution of hepatocyte cell surface in animals treated with si-Itgb1 for 10 weeks. Cell surface was assessed on phalloidin-stained liver sections (~100 cells per animal) using ImageJ software ( n =4 per group). ( e ) Effect of long-term (10 weeks) knockdown of Itgb1 on hepatocyte apical domains (canaliculi) in adult mice treated with si-Itgb1 for 10 weeks. Arrows indicate distorted canaliculi. Scale bar, 50 μm. ( f ) Increased abundance of activated stellate cells evidenced by immunofluorescent staining for α-smooth muscle actin (α-Sma). Scale bar, 100 μm. Full size image Given the alterations observed under challenging conditions in vitro , we wondered whether long-term downregulation of the integrins may result in alterations in tissue organization. Indeed, deep (although incomplete) long-term knockdown of Itgb1 (longer than 7 weeks) led to significant changes in liver morphology, including (1) a distortion of morphology of bile canaliculi as evidenced by localization of Cd13 ( Fig. 3c ) and Zo1 ( Fig. 3e ), (2) a significant increase in the proportion of enlarged hepatocytes ( Fig. 3c,d ) and (3) pronounced accumulation of non-parenchymal cells, a substantial portion of which are activated myofibroblasts as judged by α-smooth muscle actin (α-Sma) staining ( Fig. 3f ). In contrast to hepatocytes, the α-Sma-positive cells remained Itgb1 positive, indicating that siRNA treatment affected primarily hepatocytes. Interestingly, TUNEL (terminal deoxynucleotidyl transferase dUTP nick end labelling) analysis did not reveal increased cell death in livers treated with siRNA against Itgb1 for 2–7 weeks ( Supplementary Fig. 4 ). 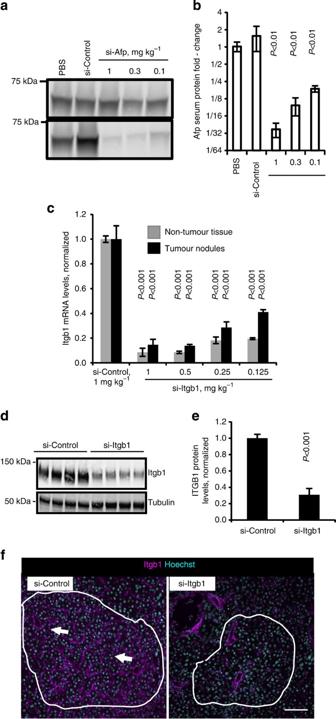Figure 4: LNP-formulated siRNA induces efficient knockdown in nodules of spontaneous hepatocellular carcinoma. (a,b) Western blot analysis of alpha-fetoprotein levels in serum samples collected form animals 10 weeks after tumour induction. Afp levels compared pre-dosing, upper panel, and 3 days after siRNA injection, lower panel (n=3, mean±s.e.m.,P-levels—comparison by the Turkeypost hoctest). (c) Dose response of Itgb1 silencing in tumour nodules and adjacent liver tissue analysed by qPCR, tissues collected 1 day after injection (n=3, mean±s.e.m., comparison by the Turkeypost hoctest). (d) Western blot analysis of Itgb1 levels in livers bearing tumours treated with si-Control of si-Itgb1 for 2 weeks. (e) Quantification of western blot, (d)n=4, mean±s.e.m., comparison by the Studentt-test. (f) Immunofluorescent staining of Itgb1 in tumour tissue (after 2 weeks of treatment with si-Itgb1). Tumour nodes countered with white dashed line. Red arrowheads indicate Itgb1 expression on tumour cells. Scale bar, 100 μm. SeeSupplementary Figs 11 and 12. Serum transaminases were only moderately upregulated after 7 weeks (no elevation after 4 weeks) of treatment with siRNA ( Supplementary Table 4 ). Together, these findings indicate that low amount (around 5–10%) of integrin subunits are sufficient to compensate pro-survival integrin signalling in normal hepatocytes at least for several weeks. These results also show that integrin knockdown has no detectable consequences for liver tissue homeostasis in the short term (2 weeks) but becomes critical on sustained downregulation. The effect of Itgb1 knockdown on spontaneous HCC The effects of Itgb1 downregulation on adult liver suggest that the function of integrins can likely be partially compensated by residual protein amounts in tissues with low rates of proliferation. Therefore, we tested whether cells with high proliferation rates may depend more critically on integrins. For this, we chose cultured mouse and human HCC cells, and found that downregulation of Itgb1 led to significant reduction in their viability and/or proliferation ( Supplementary Fig. 5a,b ). Interestingly, transfection with each of three independent sequences targeting Itgb1 led to similar decreases in cell number after 5 days of treatment ( Supplementary Fig. 5c ). To validate these results in vivo , we used a model of spontaneous HCC induced by overexpression of human MET and ΔN90-β-catenin delivered to hepatocytes by hydrodynamic injection and stably integrated into the genome by Sleeping Beauty (SB) transposase [23] , [33] , [34] . Consistent with previous publications of the model, multiple enlarged hepatocytes with altered morphology and distinct tumour nodules were observed 5 and 7 weeks after oncogene delivery, respectively. In accordance with a previous description of the model, we observed multiple enlarged hepatocytes with altered morphology at 5 weeks after oncogene delivery, and multiple foci of hepatocellular adenoma and HCC with median diameter 212 μm (25th–75th percentiles: 71–324 μm) at seven weeks ( Supplementary Fig. 6a ). At the 10th week, liver-to-body mass ratio varied from 17 to 40% versus ~5% in non-tumour control animals. Significantly increased liver-to-body mass ratio was proportional to tumour burden. Multiple tumour foci were observed per liver. Tumour nodules varied in size (from 600 to 3,000 μm) and histologically, although hyperplastic, cellular atypia and strong alpha-fetoprotein expression were prevalent ( Supplementary Fig. 6b ), markers of hepatosteatosis, local necrosis and haemorrhage were limited to only a portion of foci ( Supplementary Fig. 7 ). Strong hyperlipidaemia and hypoglycaemia were typical in tumour-bearing animals ( Table 2 ) [35] , [36] . Elevated levels of transaminases indicated pronounced hepatocyte damage ( Table 2 ). We have analysed infiltration of livers bearing HCCs by immune cells checking mRNA levels of marker genes; none of the following: Cd45 (common leukocyte antigen), Itgb2 (common chain for Cd11a,b,c and d) and Cd19 (surface protein of B-cells lineage) were elevated significantly in tumour nodules compared with livers of wild-type animals. We have used levels of Acat2, Coll1A1 and Coll1A2 mRNA as markers of stromal reaction; only collagen 1A1 was significantly upregulated (4-fold) in tumours compared with the livers of wild-type animals, indicating only miniscule stromal reaction in this model of HCC ( Supplementary Fig. 8 ), while histological analysis has not revealed any upregulation of α-Sma-positive cells in tumour or adjacent tissues. These observations are in accordance with those previously published by Stauffer et al [34] , neither apparent stromal reaction nor extensive infiltration with immune cells were observed in this model of cancer ( Supplementary Figs 9 and 10 ). Table 2 Parameters of serum chemistry in mice bearing tumours treated with si-ITGB1 for 4 weeks. Full size table siRNA delivery efficacy to late stage tumours was validated using siRNA against Afp, which is a specific marker of transformed hepatocytes ( Supplementary Figs 1e–g and 3 ) [23] . Mice at the 10th week after oncogene delivery were injected intravenously (i.v.) with Afp-specific siRNA. More than 80% knockdown of tumour marker was achieved at the dose 0.1 mg kg −1 , and >99% at 1 mg kg −1 ( Fig. 4a,b ; Supplementary Fig. 6b ). We also confirmed Itgb1 knockdown in livers bearing tumours using qPCR, western blot and immunohistochemical analysis ( Fig. 4c–f ). In tumour nodules, like in adjacent tissue, the knockdown was strong in parenchymal cells, while endothelial, activated stellate and Kupffer cells showed significant ltgb1 levels after siRNA treatment ( Supplementary Figs 11 and 12 ). Figure 4: LNP-formulated siRNA induces efficient knockdown in nodules of spontaneous hepatocellular carcinoma. ( a , b ) Western blot analysis of alpha-fetoprotein levels in serum samples collected form animals 10 weeks after tumour induction. Afp levels compared pre-dosing, upper panel, and 3 days after siRNA injection, lower panel ( n =3, mean±s.e.m., P -levels—comparison by the Turkey post hoc test). ( c ) Dose response of Itgb1 silencing in tumour nodules and adjacent liver tissue analysed by qPCR, tissues collected 1 day after injection ( n =3, mean±s.e.m., comparison by the Turkey post hoc test). ( d ) Western blot analysis of Itgb1 levels in livers bearing tumours treated with si-Control of si-Itgb1 for 2 weeks. ( e ) Quantification of western blot, ( d ) n =4, mean±s.e.m., comparison by the Student t -test. ( f ) Immunofluorescent staining of Itgb1 in tumour tissue (after 2 weeks of treatment with si-Itgb1). Tumour nodes countered with white dashed line. Red arrowheads indicate Itgb1 expression on tumour cells. Scale bar, 100 μm. See Supplementary Figs 11 and 12 . Full size image To test the effect of Itgb1 on HCC progression, we injected siRNA at 5, 6 or 8 weeks after delivery of oncogenes ( Supplementary Table 2 ). We found that weekly i.v. injections of Itgb1 siRNA for 4 and 5 weeks led to significant inhibition of HCC progression. Relative liver weights were decreased by 50% and 80%, respectively ( Fig. 5b,c ). The Itgb1 knockdown reduced expression of tumour burden marker, Afp, in the groups treated for 4 weeks (3.7-fold) and 5 weeks (110-fold) ( Fig. 5d ). It also significantly improved serum chemistry markers associated with tumour-bearing animals ( Table 2 ). Histological analysis confirmed a significant reduction in the size and number of tumour foci. Also, enlarged hepatocytes were seen in residual tumour nodules in Itgb1 siRNA-treated tumours, in contrast to control tumours ( Fig. 5e ). A second independent siRNA has demonstrated similar efficacy: >50% reduction in relative liver weight, and approximately ninefold reduction in Afp mRNA after four weekly treatments ( Supplementary Fig. 13 ). We have analysed specificity of the phenotype using simultaneous knockdown of Ago2 and Itgb1. It has been previously shown that an effect of siRNAs targeting coding sequences of mRNA is strictly dependent on activity of Ago2-slicer, and, thus, ‘on-target’ effects of such siRNAs should be diminished in the absence of Ago2, while ‘off-target’ effects are expected to persist [37] , [38] . Animals bearing tumours were treated with si-Itgb1 in combination with si-Ago2 (targeting the 3′-untranslated region and thus active even in the absence of Ago2 protein). Knockdown of Ago2 significantly decreased the efficacy of Itgb1 mRNA downregulation and blocked the effect of si-Itgb1 on HCC progression ( Supplementary Fig. 14 ). 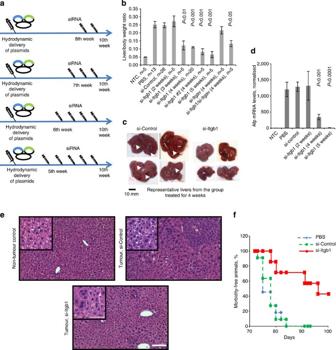Figure 5: RNAi-mediated silencing of Itgb1 reduces progression of spontaneous hepatocellular carcinoma. (a) Schematic representation of the experiment, timeline of tumour induction (injection of oncogene-encoding plasmids) and repeated injections of LNP-formulated siRNA; tissues were collected for analysis 10 weeks after the injection of plasmids. (b,c) Macroanalysis of the livers, arrowheads indicate surface tumour nodules. Liver/body mass ratio analysis, mean±s.e.m.,P-levels—comparison by the Turkeypost hocanalysis. (d) Analysis of expression of the HCC marker alpha-fetoprotein mRNA by qPCR (mean±s.e.m.P-levels—comparison by the Turkeypost hocanalysis). (e) Haematoxylin eosin staining of HCC tissue. Scale bar, 100 μm. Insets represent HCC nodules, scale bar, 50 μm. (f) Kaplan–Meier analysis of a morbid-free time after delivery of plasmids encoding oncogenes treated with PBS, control or anti-Itgb1 siRNA,n=8–10 (P<0.002, logrank test). NTC, non-tumour control mice. Figure 5: RNAi-mediated silencing of Itgb1 reduces progression of spontaneous hepatocellular carcinoma. ( a ) Schematic representation of the experiment, timeline of tumour induction (injection of oncogene-encoding plasmids) and repeated injections of LNP-formulated siRNA; tissues were collected for analysis 10 weeks after the injection of plasmids. ( b , c ) Macroanalysis of the livers, arrowheads indicate surface tumour nodules. Liver/body mass ratio analysis, mean±s.e.m., P -levels—comparison by the Turkey post hoc analysis. ( d ) Analysis of expression of the HCC marker alpha-fetoprotein mRNA by qPCR (mean±s.e.m. P -levels—comparison by the Turkey post hoc analysis). ( e ) Haematoxylin eosin staining of HCC tissue. Scale bar, 100 μm. Insets represent HCC nodules, scale bar, 50 μm. ( f ) Kaplan–Meier analysis of a morbid-free time after delivery of plasmids encoding oncogenes treated with PBS, control or anti-Itgb1 siRNA, n =8–10 ( P <0.002, logrank test). NTC, non-tumour control mice. Full size image Injection of si-Itgav did not have any effect on tumour progression either alone or in a combination with si-Itgb1 ( Fig. 5b ; Supplementary Fig. 13 ), suggesting that only signals from integrin receptors comprising β1 subunits are critical for the HCC progression. We also confirmed that treatment of HCC-bearing animals with si-Itgb1 did not induce a significant inflammatory reaction compared with control siRNA as evidenced by measuring levels of mRNA of immune cell markers, including Cd45, Cd19 and Itgb2 or cytokines Il1b, 6, Inf1b, Ifnγ and Tnf-α. Immunohistochemical staining of tumour tissues has not revealed change in overall number of Kuppfer cells or monocytes in tumour tissues treated with si-Itgb1 both short term as well as after 2 weeks of treatment ( Supplementary Figs 9 and 10 ). On the other hand, we have tested whether the observed phenotype can be explained by depletion of activity of macrophages. We have treated tumour-bearing animals for 4 weeks with clodronate liposomes (weekly injections); this treatment has not revealed any change in tumour progression ( Supplementary Fig. 15 ). These data suggest that the effect of siRNA-mediated knockdown of Itgb1 on the progression of HCC is not mediated by modulation of immune response. We performed the Kaplan–Meier analysis for animals treated with Itgb1 siRNA and control siRNA ( Fig. 5f ). Itgb1 siRNA-treated mice had significantly longer morbidity-free survival ( P <0.002, logrank test). Median morbidity-free survival was 74.5, 75 and 95 days for groups treated with phosphate-buffered saline (PBS), control and specific siRNA, respectively. To demonstrate the effect of Itgb1 on tumour cell proliferation and survival, we used Ki67 staining as a marker of cellular proliferation ( Fig. 6a ). In the animals treated with control siRNA, Ki67-positive cells (23.6±5.0%) were located mainly in the tumour foci. Itgb1 knockdown for 4 weeks led to a significant reduction in Ki67-positive cells (6.6±2.4%, P <0.05, Student’s t -test). Expression levels of genes associated with cell cycle progression were reduced in Itgb1 siRNA-treated tumours compared with control siRNA-treated tumours, for example, Cclna1 and Cclnd1 ( Fig. 6e ). Positive TUNEL staining was increased in HCC foci of animals treated with Itgb1 siRNA for 2 weeks ( Fig. 6b ). Cleaved caspase 3 (p17) was significantly upregulated in tumour-bearing livers of mice treated with Itgb1 siRNA ( Fig. 6c,d ) indicating elevated apoptosis on downregulation of Itgb1 expression. Analysis of gene expression revealed significantly upregulated mRNA levels of genes associated with cell death, for example, Gas2l3, Ckap2, Gadd45B, Cdkn3 and reduced levels of genes associated with cell survival, for example, Birc2 ( Fig. 6e ). Our results suggest that integrin β1 expression is essential for HCC progression and survival. 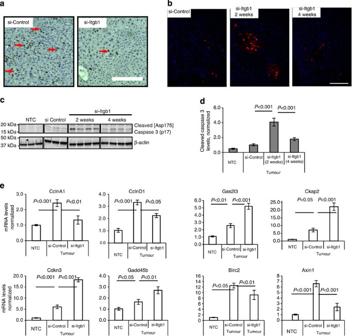Figure 6: Effect of Itgb1 silencing on proliferation and survival of tumour cellsin vivo. (a) Ki67 staining was used to analyse proliferation of tumour cells, brown nuclei indicate positive cells (arrowheads). Scale bar, 200 μm. (b) Analysis of cell death in tumour nodules by terminal deoxynucleotidyl transferase dUTP nick end labelling (TUNEL), red nuclei represent TUNEL-positive cells. Scale bar, 200 μm. (c,d) Analysis of expression of cleaved caspase 3 (p17) in livers bearing tumours and treated with either control or Itgb1 siRNA (n=3–4, means±s.e.m., comparison by the Turkeypost hoctest). For Itgb1 knockdown validation seeFig. 8a, (e) qPCR analysis of expression of Cclna1, Cclnd1, Gas2l3, Ckap2, Cdkn3, Gadd45b, Birc2 and Axin2 (n=5–6, mean±s.e.m., comparison by the Turkeypost hoctest). NTC, non-tumour control mice. Figure 6: Effect of Itgb1 silencing on proliferation and survival of tumour cells in vivo . ( a ) Ki67 staining was used to analyse proliferation of tumour cells, brown nuclei indicate positive cells (arrowheads). Scale bar, 200 μm. ( b ) Analysis of cell death in tumour nodules by terminal deoxynucleotidyl transferase dUTP nick end labelling (TUNEL), red nuclei represent TUNEL-positive cells. Scale bar, 200 μm. ( c , d ) Analysis of expression of cleaved caspase 3 (p17) in livers bearing tumours and treated with either control or Itgb1 siRNA ( n =3–4, means±s.e.m., comparison by the Turkey post hoc test). For Itgb1 knockdown validation see Fig. 8a , ( e ) qPCR analysis of expression of Cclna1, Cclnd1, Gas2l3, Ckap2, Cdkn3, Gadd45b, Birc2 and Axin2 ( n =5–6, mean±s.e.m., comparison by the Turkey post hoc test). NTC, non-tumour control mice. Full size image MET and β-catenin expression and signalling To assess the early effects of Itgb1 knockdown on expression and signalling of oncogenes driving tumour growth, we compared the expression of MET and β-catenin in animals treated for 2 and 4 weeks with Itgb1 siRNA. Antibodies against β-catenin recognize both endogenous mouse (~90 kDa) and human ΔN90-β-catenin (~80 kDa). Exogenous β-catenin in tumour-bearing livers was expressed about threefold higher than the endogenous protein in the livers of non-tumour control animals, while endogenous protein levels were not changed ( Fig. 7a,b ). After treatment for 2 weeks with Itgb1 siRNA, tumour burden was not changed and transgene expression was not significantly altered. In the group treated for 4 weeks, expression of ΔN90-β-catenin was reduced (mRNA by 1.8-fold ( Fig. 7d ), protein by 1.6-fold). Itgb1 siRNA treatment also reduced phosphorylation of β-catenin (S625), likely reducing transcriptional activity, which was exemplified by Axin1 mRNA levels ( Fig. 6e ). 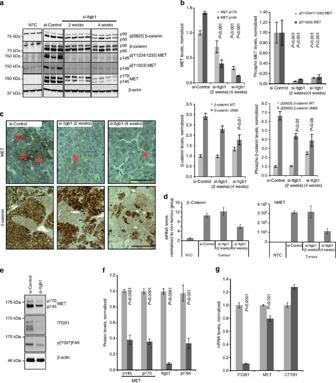Figure 7: Effect of Itgb1 downregulation on MET signalling and expression in mouse HCC. (a) Analysis of expression and phosphorylation of MET and β-catenin in tumour tissues treated with siRNA. (b) Western blot (a) quantification (n=3–4, means±s.e.m., comparison by the Turkeypost hoctest). For Itgb1 knockdown validation seeFig. 8a. (c) Immunohistochemical analysis of expression of MET and β-catenin in tumour nodules. Scale bar, 100 and 400 μm, correspondingly. Arrowheads indicate cytoplasmic and arrows indicate membrane expression of MET. (d) Analysis of hβCatenin and hMET oncogenes mRNA levels by qPCR (n=5.P-levels—comparison by the Turkeypost hoctest, versus the si-Control-treated group. (e) Expression of MET, ITGB1 and phosphorylated FAK in Hep3B cells treated with siRNA. (f) Quantification of (e), 4–6 independent transfections were analysed, mean±s.e.m.,P-levels—comparison by the Studentt-test. (g) Confirmation of ITGB1 mRNA knockdown and MET and CTTB1 mRNA levels in Hep3B cells by qPCR, mean±s.e.m.,P-levels—comparison by the Studentt-test. NTC, non-tumour control mice. Light grey, si-Control treated; dark grey, si-Itgb1-treated cells. Figure 7: Effect of Itgb1 downregulation on MET signalling and expression in mouse HCC. ( a ) Analysis of expression and phosphorylation of MET and β-catenin in tumour tissues treated with siRNA. ( b ) Western blot ( a ) quantification ( n =3–4, means±s.e.m., comparison by the Turkey post hoc test). For Itgb1 knockdown validation see Fig. 8a . ( c ) Immunohistochemical analysis of expression of MET and β-catenin in tumour nodules. Scale bar, 100 and 400 μm, correspondingly. Arrowheads indicate cytoplasmic and arrows indicate membrane expression of MET. ( d ) Analysis of hβCatenin and hMET oncogenes mRNA levels by qPCR ( n =5. P -levels—comparison by the Turkey post hoc test, versus the si-Control-treated group. ( e ) Expression of MET, ITGB1 and phosphorylated FAK in Hep3B cells treated with siRNA. ( f ) Quantification of ( e ), 4–6 independent transfections were analysed, mean±s.e.m., P -levels—comparison by the Student t -test. ( g ) Confirmation of ITGB1 mRNA knockdown and MET and CTTB1 mRNA levels in Hep3B cells by qPCR, mean±s.e.m., P -levels—comparison by the Student t -test. NTC, non-tumour control mice. Light grey, si-Control treated; dark grey, si-Itgb1-treated cells. Full size image Antibodies against MET recognize only exogenous protein (human MET, hMET): a major 145-kDa band corresponds to the mature protein, and a minor 170-kDa band is an immaturely glycosylated form ( Fig. 7a,b ) [39] . The treatment with Itgb1 siRNA for 2 weeks slightly reduced p170, reduced p145 about 3.6-fold and did not significantly change mRNA levels of hMET ( Fig. 7d ). The treatment for 4 weeks reduced p170 expression threefold and p145 expression ~10-fold, while hMET mRNA was reduced about threefold ( Fig. 7d ). It is noteworthy that p170 became the predominant form of MET even after the brief 2-week treatment with Itgb1 siRNA. These results indicate that loss of integrin expression causes a reduction in MET protein maturation, leading to decrease in total MET content. Consistently, immunohistochemical analysis revealed a marked reduction in MET expression in Itgb1 siRNA-treated animals. Cytoplasmic and membrane expression was obvious in tumour foci in animals treated with control siRNA, whereas weak diffuse cytoplasmic expression was observed in animals treated with Itgb1 siRNA for both 2 and 4 weeks ( Fig. 7c ). We analysed phosphorylation of MET Y1234/Y1235 as a reporter of its kinase activity [40] . Treatment with Itgb1 siRNA markedly reduced both MET phosphorylation and total protein levels ( Fig. 7a,b ). On the basis of these results, we hypothesized that si-Itgb1 retards MET protein maturation acting directly on tumour cells. To test this hypothesis, we analysed the effect of Itgb1 siRNA on endogenous MET expression in HCC cells (Hep3b). Western blot analysis confirmed a 60% reduction in MET expression in cells treated with Itgb1 siRNA along with ~90% knockdown of ITGB1 protein and ~60% reduction in FAK phosphorylation, while changes in MET mRNA levels were minimal ( Fig. 7e–g ). These results were confirmed with a second siRNA targeting a non-overlapping region of Itgb1 ( Supplementary Fig. 16a ). Similar results were obtained using human colorectal carcinoma cells (HT29) and primary human melanocytes ( Supplementary Fig. 16b–d ). Co-immunoprecipitation analysis showed that the mature MET (p145) was co-precipitated with ITGB1 and vice versa mature ITGB1 was co-precipitated MET antibodies ( Supplementary Fig. 17 ). We next asked which signalling pathways are activated in the MET/ΔN90-β-catenin model of HCC and whether Itgb1 knockdown affects pathway activation. Phospho-specific antibodies identified elevated levels of active forms of the following signalling molecules in tumour-bearing livers: Egfr, Erk1/2 and Stat3. Following two weekly treatments with Itgb1 siRNA, phosphorylation levels of each of these molecules were reduced ( Fig. 8 ). Furthermore, tumour burden is correlated with overexpression of Egfr. Phosphorylation of Fak serves as a marker of Itgb1 clustering and activity [41] . After two treatments with Itgb1 siRNA, Fak Y397 phosphorylation was significantly reduced, as were levels of Egfr that is an additional marker of tumour burden. Altogether, these results suggest that Itgb1 knockdown causes a strong reduction in MET signalling pathway, consisting with its effects on tumour progression. 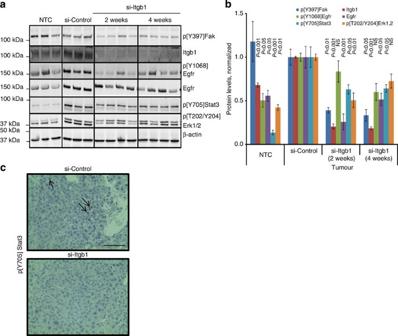Figure 8: siRNA against Itgb1 reduces overactivation of various signalling pathways in spontaneous liver tumour. (a) Western blot analysis of tumour tissues treated by control siRNA. (b) Quantification of the western blot (a) (n=3–4, means±s.e.m., comparison by the Turkeypost hoctest). (c) Immunohistochemical analysis of phosphorylated Stat3 expression in the liver tissues (arrows indicate positively stained nuclei). Scale bar, 100 μm. NTC, non-tumour control mice. Figure 8: siRNA against Itgb1 reduces overactivation of various signalling pathways in spontaneous liver tumour. ( a ) Western blot analysis of tumour tissues treated by control siRNA. ( b ) Quantification of the western blot ( a ) ( n =3–4, means±s.e.m., comparison by the Turkey post hoc test). ( c ) Immunohistochemical analysis of phosphorylated Stat3 expression in the liver tissues (arrows indicate positively stained nuclei). Scale bar, 100 μm. NTC, non-tumour control mice. Full size image Mouse hepatocytes express integrins, including α1β1, α5β1, α9β1, αvβ1 and αvβ5. Acting as receptors for ECM components, integrins are postulated to be key regulators of cell function. Using an in vivo RNAi approach, we could demonstrate for the first time knockdown of all integrin receptors in hepatocytes that impaired binding of isolated hepatocytes to matrices. The application of siRNA formulated into nanoparticles conferred significant advantages comparing with classical genetic approaches, including flexibility of experimental design, ability to manipulate the expression of several genes without animal breeding and translational potential. Given the previously reported effects of integrin inhibition on cell viability and morphology in tissue culture studies, it was expected that integrin knockdown in the mouse liver would have consequences for cell survival and tissue integrity. Significant effects on hepatocyte morphology were observed after extended treatment with Itgb1 siRNA (after 7 weeks), which includes alterations in cell morphology, hepatocyte hypertrophy and apical distortion. However, even after extended siRNA treatment (10 weeks maximum), no significant effect on hepatocyte viability was detected. Interestingly, upregulation of transcription of other integrin family members, or collagen receptors (for example, Ddr1), was not observed. The effect of sustained integrin knockdown on the hepatocyte size is consistent with the results obtained on Itgb1 knockdown during liver regeneration [27] and previously observed effects of integrin-blocking peptides on perfused liver [42] , [43] , revealing the importance of integrin-dependent signalling on hepatocyte swelling and osmoregulation. Our results show that under challenging conditions of in vitro culturing of hepatocytes, integrins are important for cell adhesion, polarity and cell–cell interaction. The low residual levels of integrins in liver treated with specific siRNAs may likely be sufficient to maintain integrity of the mature pre-formed tissue in vivo during the treatment for at least several weeks. This hypothesis is supported by findings of Speicher et al. [27] demonstrating that short-term Itgb1 knockout resulted in increased transaminase activities in the serum, suggesting that even acute complete loss of integrin signalling leads to hepatocyte damage. Long-term knockdown of integrins’ expression leads to more pronounced alterations in liver morphology, reflecting most likely the slow proliferation rate of hepatocytes [44] , [45] . To test the effects of in vivo RNAi-mediated Itgb1 inhibition on transformed hepatocytes, we employed a MET/ΔN90-β-catenin-driven mouse model of HCC in which relatively rapid tumour progression occurs in fully immunocompetent mice. Mosaic transformation of hepatocytes by MET and ΔN90-β-catenin using SB transposase mimics the aetiology of a subset of human HCC [23] , a cancer with limited treatment options and very poor prognosis [46] . Studies in a tet-regulated MET model of HCC have shown that switching off MET expression leads to reduced proliferation and increased apoptosis of tumour cells. Moreover, ECM interaction has been shown to be important for MET signalling [15] . Beta-catenin is another oncogene frequently activated in HCC. Mutations in the amino terminus of β-catenin inhibit regulation by the tumour suppressive antigen-presenting cell complex, and allow the protein to enter the nucleus and activate pro-oncogenic targets [47] . We have demonstrated efficient delivery of formulated siRNA to tumour nodules in the MET/ΔN90-β-catenin-induced tumour model. We have not observed any elevated immune response to si-Itgb1 compared with treatment with control siRNA, these findings, together with previous observations as well as characterization of knockdown specificity, strongly suggest that the phenotype is cell autonomous and results from knockdown of Itgb1 in tumour cells [24] , [48] . Our data suggest that the effect of Itgb1 knockdown on HCC progression is at least partially mediated by regulation of MET protein levels and its signalling activity. siRNA-mediated knockdown of Itgb1 reduces phosphorylation of MET and inhibits protein maturation without affecting its mRNA levels. These results are observed both in vivo in mouse model of HCC and in vitro in human HCC. Previously, interaction of MET and integrin α5 subunit and integrin β4 subunit has been demonstrated by co-immunoprecipitation; here, we demonstrate its interaction with integrin β1 at least in Hep3B cells [49] , [50] . Reduction in phosphorylation of Stat3 may serve as an additional evidence of downregulation of MET signalling on treatment with siRNA. We have also demonstrated that Itgb1 silencing reduces β-catenin phosphorylation, which is predicted to blunt its transactivation function. A range of signalling proteins are changed in HCC overexpressing MET/ΔN90-β-catenin, including overexpression of Egfr. Although lowering of Itgb1 partially decreases levels of this protein, the effect is much less profound compared with reduction in mature MET. Lee et al. [51] has recently reported that knockdown of CSN5 using siRNA was efficient in decreasing HCC growth in vivo (xenograft model) and in vitro due to downregulation of transcriptional activity of MYC, that is, reduction in their target genes, including Itgb1. In our model, we have not observed any notable change in Myc expression in response to knockdown of Itgb1. The net effect of siRNA-mediated Itgb1 inhibition is to significantly inhibit tumour proliferation and increase tumour cell apoptosis resulting in extended morbidity-free survival of tumour-bearing mice. Integrins have long been investigated as therapeutic targets in a variety of diseases, including cancer. Contrary to other methods of integrin inhibition, including antibodies and antagonistic peptides, siRNA-mediated gene silencing leads both to downregulation of integrin signalling and to elimination of membrane and intracellular fractions of integrin, blocking its ability to serve as a binding platform and lowering of all ligand-independent actions of integrin receptors [16] . It is important to note that normal hepatocytes can, at least partially, adapt to decreased level of integrin signalling, in contrary to cancer cells, isolated cells in vitro (this study) and proliferating hepatocytes in the regenerating liver (study by Speicher et al. [27] ). Inhibition of integrin receptors comprised with Itgav subunit is often reported as efficient anti-tumour therapy acting both directly on the cancer cells and as an anti-angiogenic factor [16] . Interestingly, we do not observe any effect of knockdown of Itgav either in normal liver or in HCC. These findings, collectively with others, indicate high therapeutic potential of anti-Itgb1 siRNA. In light of the findings that inhibition of Itgb1 signalling may increase tumour sensitivity to irradiation and chemotherapy, Itgb1-specific siRNA may be suggested as part of a combinatorial therapy [22] , [52] . siRNA description and LNP formulation Twenty-eight siRNAs targeting both human and mouse ITGB1 sequence (NCBI Genbank accession codes NM_010578.2 , NM_002211.3 , NM_133376.2 , NM_033668.2 ), 24 siRNAs targeting mouse Itgav sequence (NCBI Genbank accession code NM_008402.2 ) and 47 siRNAs targeting mouse Afp sequence (NCBI Genbank accession code NM_007423.4 ) with the lowest off-target potential were bioinformatically selected as previously described [24] . siRNA were synthesized at Alnylam Pharmaceuticals Inc. as previously described [26] . Modified bases (2′OMe) were incorporated into an oligoribonucleotide chain using standard phosphoramidite chemistry. Phosphorothioate linkages were introduced by replacement of the iodine oxidizer solution with a solution of the Beaucage reagent in acetonitrile (1%). Sets of siRNA targeting ITGB1, Itgav and Afp were screened as described elsewhere [24] using NIH3T3 and Hep3B, Hepa1-6 and Hepa1c1c7. respectively. siRNA with the lowest half-maximal inhibitory concentration were selected ( Supplementary Table 5 ) Chemical modifications were introduced to stabilize siRNA in vivo , reduce off-target potential of the sense strand and minimize immune response. LNP with siRNA were formulated as previously described. Briefly, ionizable lipid or cationic lipid, disteroylphosphatidyl choline, cholesterol, and 1,2-dimyristoyl-sn-glycerol, methoxypolyethylene glycol at a molar ratio of ~50/10/38.5/1.5 were mixed with siRNA to allow spontaneous particle formation [25] , [53] , [54] . The particles mean diameter was ~70 nm. Cell culture HCC cells p53−/−;MYC was provided by Dr Scott Lowe and Dr Xue Wen [55] ; HCC cells overexpressing hMET and β-Catenin were derived from mice in our laboratory; HCC Hep3B and colorectal carcinoma HT29 obtained from ATCC were propagated in Dulbecco’s modified Eagle’s medium supplemented with 10% fetal bovine serum and adult melanocyte (NHEM-Ad) cell from Lonza were grown using the MGM-4 Bulletkit supplemented with endothelin. Two latter cell types were selected for in vitro experiments based on relative levels of MET expression and effect of cell attachment on MET levels [15] . All cells were grown on BD BioCoat collagen I-coated plasticware. Cells were transfected with siRNA using either Lipofectamine RNAiMAX (Invitrogen) or LNP with siRNA as described elsewhere [24] . Confirmation of the RNAi mechanism To validate RNAi mechanism of mRNA downregulation, we have used an established method 5′RACE [26] : wild-type mice were injected with specific (si-Itgb1) or control siRNA (three animals per group), liver tissues were harvested and snap-frozen 6 h post injection. To validate mechanism of siRNA-mediated mRNA reduction in HCC, we have collected tumour tissues (established nodules 60 days after oncogene delivery) at 24 h after siRNA injection (si-Afp). The 5′RACE was performed on isolated total RNA according to the manufacture’s protocol (Generacer kit, Invitrogen). Primers used for the 5′RACE are listed in ( Supplementary Table 6 ). Animals C57BL/6 and FVB/N mice were purchased from Charles River laboratories, Balb/cJ mice were purchased from JAX laboratories. All animals received humane care, and study protocols were approved by the Committee on Animal Care of MIT and Institutional Animal Care and Use Committee of Alnylam Pharmaceutical certified by the American Association for Accreditation of Laboratory Animal Care. Animals were maintained in a conventional barrier animal facility with a climate-controlled environment on a 12-h light/12-h dark cycle, fed ad libitum with regular rodent chow. Schematic presentation of in vivo experiments is summarized in Supplementary Table 2 . Experiments with adult animals. Seven to nine-week-old mice received either PBS or siRNA in LNP formulations at various concentrations via tail vein injection (i.v.). Animals received either one injection or two injections once per week ( Supplementary Table 2 ). Knockdown of Itgb1 and Itgav was tested with C57BL/6 and FVB/n mice, and Afp knockdown was tested in Balb/cJ strain [56] . Blood for analysis was collected from retro-orbital sinus under isoflurane anaesthesia. Animals were killed by CO 2 overdose; tissues were harvested at different time points as indicated. Experiments with growing mice. Timed-pregnant FVB/N mice (confirmed pregnancy at shipping) were purchased from Charles River Laboratories, new born mice were injected intraperitoneally starting from day 7 every third day with either PBS- or LNP-formulated siRNA 10 ml kg −1 0.5 mg kg −1 for 3 weeks ( Supplementary Table 2 ). HCC induction and treatment with siRNA. Plasmids encoding human ΔN90-β-catenin, human MET and SB transposase were kindly provided by Dr Xin Chen (UCSF, San Francisco, CA) [23] . Plasmids with low endotoxin contamination (<5 EU mg −1 , prepared by Aldveron) were hydrodynamically injected into 7–8-week-old FVB/N mice as previously described. To confirm efficient knockdown of genes in the liver tumour, we have used Afp as a selective marker. A specific siRNA against Afp formulated into LNP was injected i.v. once at the 9th week after plasmid delivery. Animals were euthanized at 72 h post injection. Serum for analysis and liver pieces for histology and immunohistochemistry were collected; the rest of the liver was ground and aliquots of tissue powder were used for protein and mRNA analysis. LNP-formulated siRNAs against integrins were injected once per week (1 mg kg −1 ) as indicated. Animals were euthanized after 2–5 injections of siRNA. To assess the ability of Itgb1 siRNA to slow down HCC progression, we have started treatment of animals at the 7th week post tumour induction; animals received one weekly injection of siRNA. Animals were euthanized when following signs of morbidity were observed: significant weight loss (>20%), hair loss, dehydration, inability to move, feed, groom and defecate. Two researchers observed animals daily and consensus decision was made for each mouse. Isolation and analysis of primary hepatocytes Hepatocytes were isolated from C57BL/6 mice via collagenase perfusion as described previously [57] . To assess hepatocyte repolarization, cells were plated in collagen gel-coated 24-well plates at 200,000 cells per well in Williams E medium (Lonza), substituted with 10% fetal bovine serum, 100 nM dexamethasone and penicillin/streptomycin and maintained at 37 °C in an atmosphere with 5% CO 2 and cultured under conditions for maintenance of cell polarity and liver-specific metabolic functions [58] . To analyse Itgb1 expression in hepatocytes, cells were incubated with either anti-ITGB1 or isotype control antibodies labelled with Alexa647 and analysed using flow cytometry. Residual contamination of hepatocytes by endothelial cells (the second major population of liver cells) was assessed by comparison of relative levels of specific marker—Tek (Tie2) to hepatocyte-specific gene ( Apoc3 ). To analyse adhesion of hepatocytes CytoSelect 48-Well Cell Adhesion Assay (Cells Biolabs) was used according to the manufacturer’s protocol. Histological and immunocytochemical analysis Freshly collected tissues were fixed in 4% buffered paraformaldehyde and embedded into paraffin. Five-micrometre-thick sections were subjected to hematoxylin eosin staining or immunohistochemistry. Envision system (Dako) was used for indirect peroxidase reaction using DAB as chromogen. Primary antibodies used are listed in Supplementary Table 7 . Immunofluorescent analysis was performed using 5 μm frozen sections post-fixed with 2% buffered paraformaldehyde. Cells were fixed with 2% buffered paraformaldehyde solution and permeabilised with 1% Triton X-100 in PBS. Secondary antibodies labelled with Alexa 488, Alexa 555 and Alexa 647 (Invitrogen) were used to visualize antigen localization. TUNEL staining was performed on liver sections treated with proteinase K using the In Situ Cell Death Detection Kit, TMR red (Roche). Immunoprecipitation and Western blots Aliquots of ground liver tissue were homogenized in radioimmunoprecipitation assay (RIPA) buffer with inhibitors of proteases and phosphatases (Thermo Fisher), cells were washed with cold PBS and lysed in same RIPA buffer, 10–50 μg of total protein was resolved on TGX gradient gels (Bio-Rad), transferred to nitrocellulose membranes and incubated with various antibodies ( Supplementary Table 7 ). For immunoprecipitation, 1 mg of protein lysate (500 μl) was incubated overnight (4 °C) with recommended dilution of antibodies, protein A sepharose was used to pull down the complexes, pellet was washed three times with ice cold RIPA and resuspended in βME-loading buffer. Secondary antibodies labelled with infrared fluorophores (IRDye680 or IRDye780) (Lycor) were used to visualize protein bands. Membranes were scanned on an Odyssey Scanner and images were quantified with ImageJ as described online ( http://lukemiller.org/index.php/2010/11/analyzing-gels-and-western-blots-withimage-j/ ). Full-scan images of representative western blots are shown in Supplementary Fig. 18 . Flow cytometry Isolated hepatocytes or collected cultured cells (grown on collagen I and detached using 0.25% collagenase solution) were incubated with antibodies labelled with fluorophores (Biolegend, Supplementary Table 7 ) or appropriate isotype control and analysed on FACS LSR II (BD Biosciences). Data were analysed using FlowJo 7.8 (TreeStar Inc.). Gene expression analysis Levels of mRNAs were assessed by branched DNA assay (Affymetrix) or qPCR using Roche LightCycler 480. Gapdh, β-actin mRNA and 18S rRNA were used as housekeeping controls. The mRNA levels were normalized to the level of housekeeping gene and to an average value of control group. Specific probes and primers are listed in Supplementary Table 8 . Serum chemistry Albumin, high-density lipoprotein, low-density lipoprotein, direct bilirubin, aspartate aminotransferase, alanine transaminase and total bile acids were measured in serum using Beckman Coulter reagents and the Olympus Au400 autoanalyser. Statistical analysis For multiple comparisons, one-way analysis of variance followed by a Turkey post hoc test was performed. A two-tailed Student’s t -test was used for individual comparisons. GraphPad Prism 5 package was used. How to cite this article: Bogorad, R. L. et al. Nanoparticle-formulated siRNA targeting integrins inhibits hepatocellular carcinoma progression in mice. Nat. Commun. 5:3869 doi: 10.1038/ncomms4869 (2014).